Ultrafast acousto-plasmonic control and sensing in complex nanostructures Coherent acoustic phonons modulate optical, electronic and mechanical properties at ultrahigh frequencies and can be exploited for applications such as ultratrace chemical detection, ultrafast lasers and transducers. Owing to their large absorption cross-sections and high sensitivities, nanoplasmonic resonators are used to generate coherent phonons up to terahertz frequencies. Generating, detecting and controlling such ultrahigh frequency phonons has been a topic of intense research. Here we report that by designing plasmonic nanostructures exhibiting multimodal phonon interference, we can detect the spatial properties of complex phonon modes below the optical wavelength through the interplay between plasmons and phonons. This allows detection of complex nanomechanical dynamics by polarization-resolved transient absorption spectroscopy. Moreover, we demonstrate that the multiple vibrational states in nanostructures can be tailored by manipulating the geometry and dynamically selected by acousto-plasmonic coherent control. This allows enhancement, detection and coherent generation of tunable strains using surface plasmons. Plasmonic nanostructures have revolutionized nano-optics [1] , [2] , [3] with their ability to generate strong localized electromagnetic fields when illuminated from the far-field, analogous to antennas for light [4] . The generation, detection and control of ultrahigh frequency phonons have been a topic of intense research [5] , [6] , [7] , [8] , [9] , [10] . Plasmons are effective for localizing light in a subwavelength volume and are ideal candidates for manipulating nanoscale mechanical motion because of their large absorption cross-sections, subwavelength field localization and high sensitivity to geometry and refractive index changes. This efficient absorption makes the plasmon an effective transducer of far-field radiation into phonons [5] : the plasmonic nanostructure absorbs energy from the laser pulse and rapidly expands, generating coherent acoustic phonons through impulsive thermal excitation [11] , [12] , [13] , [14] . When a metallic nanostructure first absorbs an ultrashort laser pulse, a localized surface plasmon, a coherent oscillation of electrons, is excited. The electrons rapidly dephase on a 5- to 20-fs timescale because of electron–electron scattering, electron–surface scattering and radiation damping [15] . The electrons then superdiffuse throughout the nanostructure at the Fermi velocity (~10 6 m s −1 ), distributing their kinetic energy over the nanostructure within ~100 fs (ref. 16 ). The electrons transfer energy to the lattice, resulting in a rapid thermal expansion of the structure that sets off oscillations between the initial and expanded lattice spacing, known as coherent acoustic phonons. The phonons can be detected afterwards with a weak probe pulse that senses the phonons through the strain-induced shift of the plasmon resonance [6] . Opto-mechanical resonators allow strong light–matter interactions at increasingly smaller scales. Micron-scale dielectric resonators allow single-photon control of opto-mechanical properties [17] , tunable electromagnetically induced transparency [18] and quantum-coherent coupling between light and mechanical modes [19] . Unique plasmonic dispersions allow researchers to investigate acoustic modes at subwavelength scales in simple structures such as spheres and bars [6] . Plasmonic nanoparticles offer the benefits of higher absorption, thus more efficient phonon excitation through impulsive thermal expansion, and higher detection sensitivity than equivalently sized dielectric nanoparticle because of their resonant nature and the large photoelastic coefficient of metal [20] . These characteristics allow phonon excitation and detection in nanostructures containing only hundreds of atoms [21] . Through electromagnetic coupling, larger nanoantennas have been used to enhance the phonon detection in adjacent smaller nanoparticles [22] . Recent advances in spatial control of surface plasmons from the far field have the potential to allow selective subwavelength detection of phonon modes—previously only possible using an X-ray free-electron laser [9] . Here we show that in a multimodal nanostructure (plasmonic and phononic), manipulating the polarization of the probe laser allows dynamic control over the region in which mechanical motion is detected. We demonstrate selective excitation and detection of mechanical motion of plasmonic nanostructures through the design of the particle’s geometry and time domain-coherent control. Acousto-plasmonic resonators To demonstrate the capabilities of plasmons for nanoscale detection and manipulation of phonons, we designed and fabricated nano Swiss-cross samples ( Fig. 1a ) that exhibit localized phonon modes. The phonon modes of a metal nanostructure are high-frequency mechanical distortions of the metallic lattice and are the solutions of the Navier equation with continuity of displacement and stress at the nanostructure boundaries [21] . The displacement profile for the two lowest-order phonon modes of a Swiss-cross are shown in Fig. 1b,c . The mode in which the two arms oscillate in phase is the symmetric mode and the mode where the arms oscillate out of phase is the antisymmetric mode. These modes can be viewed as the hybridization of the extensional modes of the two arms. The modes are symmetric and antisymmetric in the context of coupled mode theory and not in terms of spatial symmetry [23] , [24] . The phonons modify the optical properties of a nanostructure through mechanical distortion of the geometry and strain-induced modifications [20] of the refractive index of the metal. The two contributions to the optical response are of the same order of magnitude. 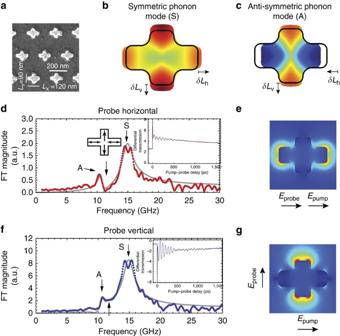Figure 1: Selective phonon detection. The 120 × 90 nm Swiss-cross nanostructures (a) support two mechanical eigenmodes, the symmetric eigenmode (b), in which the two arms oscillate in phase, and the antisymmetric (c), where the two arms oscillate out of phase.b,care simulated mechanical displacement profiles at the eigenfrequencies. The superposition between the modes dictates the mechanical dynamics, whose phase and amplitude can be detected with localized surface plasmon polaritons. Each probe plasmon polarization yields a projection of the dynamics, allowing us to sense the mechanical displacement along each axis. The phonon strains the nanostructure, causing geometry and refractive index changes, which in turn modulate the plasmonic resonance, allowing the phonon to be detected through transient optical transmission spectroscopy. The simulated electric field magnitude is plotted for the plasmons excited by a horizontal (e) and vertical probe pulse (g). The Fourier transform of the transient transmission for a (d) horizontally polarized probe and a (f) vertically polarized probe. The interference effect at 11 GHz in the transient transmission spectrum for a horizontally polarized probe pulse (d) originates from the two phonon modes changing the optical transmission with equal magnitude and opposite signs, resulting in a zero signal in the differential transmission. When the probe polarization is vertical (f), the two phonon modes affect the transmission with the same sign, resulting in a constructive contribution (seeSupplementary Fig. 10for the phase of the FT). The grey curves ind,fare fits with two phonon modes of varying sign using the fit function inSupplementary Note 1. Figure 1: Selective phonon detection. The 120 × 90 nm Swiss-cross nanostructures ( a ) support two mechanical eigenmodes, the symmetric eigenmode ( b ), in which the two arms oscillate in phase, and the antisymmetric ( c ), where the two arms oscillate out of phase. b , c are simulated mechanical displacement profiles at the eigenfrequencies. The superposition between the modes dictates the mechanical dynamics, whose phase and amplitude can be detected with localized surface plasmon polaritons. Each probe plasmon polarization yields a projection of the dynamics, allowing us to sense the mechanical displacement along each axis. The phonon strains the nanostructure, causing geometry and refractive index changes, which in turn modulate the plasmonic resonance, allowing the phonon to be detected through transient optical transmission spectroscopy. The simulated electric field magnitude is plotted for the plasmons excited by a horizontal ( e ) and vertical probe pulse ( g ). The Fourier transform of the transient transmission for a ( d ) horizontally polarized probe and a ( f ) vertically polarized probe. The interference effect at 11 GHz in the transient transmission spectrum for a horizontally polarized probe pulse ( d ) originates from the two phonon modes changing the optical transmission with equal magnitude and opposite signs, resulting in a zero signal in the differential transmission. When the probe polarization is vertical ( f ), the two phonon modes affect the transmission with the same sign, resulting in a constructive contribution (see Supplementary Fig. 10 for the phase of the FT). The grey curves in d , f are fits with two phonon modes of varying sign using the fit function in Supplementary Note 1 . Full size image Through their sensitivity to geometry and material properties, the surface plasmon serves as a local probe of coherent acoustic phonons. The change in probe transmission after excitation by the pump pulse is shown in the inset of Fig. 1f . The sample is an array of 35-nm-thick gold Swiss-crosses with horizontal and vertical arm lengths of 120 and 90 nm, respectively, on a quartz substrate. The transient transmission is measured using time domain spectroscopy (pump–probe) at normal incidence as discussed in the Methods section. The pump excites a plasmon that rapidly decays to non-thermalized electrons [25] . The electrons thermalize through scattering processes on a sub-picosecond timescale raising the electronic temperature and changing the interband transition rates [26] : producing a sharp peak in the transient transmission measurement [16] . The electrons then rapidly heat the lattice through electron–phonon scattering, which generates coherent acoustic phonons, the sinusoidal oscillations with a period of ~100 ps. The Fourier transform of this time trace yields the frequency response of the vibrating nanostructure: the peaks at ~10 and ~15 GHz correspond to the antisymmetric and symmetric phonon modes with quality factors of ~16 and 9, respectively. Simulations of a periodic array of Swiss-crosses on a glass substrate with no internal damping yield quality factors ( Q >500, see Supplementary Fig. 1 ) much larger than the experimentally observed quality factors, which suggests internal damping [27] , [28] , [29] and inhomogeneous broadening may contribute to the linewidth of the measured signals. Polarization-sensitive phonon detection The spatial selectivity for detecting coherent acoustic phonons, in contrast to its generation, is determined by the spatial distribution of the probe plasmon and does not depend on the electron diffusion length of the constituent materials because of the short lifetime of the probe surface plasmons. Thus, the probe plasmon can resolve strain distributions at length scales below the superdiffusion length. For the Swiss-cross, the nanostructure supports two probe plasmon modes (see Supplementary Fig. 2 for the transmission spectrum), localized in different regions of the nanostructure that can be excited with horizontal ( Fig. 1e ) and vertical polarizations ( Fig. 1g ), which enable the local detection of phonon modes. The phonon modes that create symmetric strain profiles will shift the resonance frequency of the plasmon modes polarized along both axes in the same direction. For example, the initial expansion of the nanoparticle red-shifts both the vertical and horizontal plasmon modes. In contrast, an antisymmetric phonon mode (in which a compression along one axis is accompanied by an extension along the perpendicular axis) red-shifts one plasmonic resonance while blue-shifting the other resonance. In other words, the distortions because of the symmetric and antisymmetric modes will be in phase along one axis and π out of phase along the other axis. Measuring this polarization-dependent phase allows one to determine the symmetry of the nanoscale phonon modes from a far-field measurement. We find that when the probe polarization is changed from horizontal ( Fig. 1d ) to vertical ( Fig. 1f ), a dip at 11 GHz appears. This destructive interference at 11 GHz in the transient transmission spectrum for a horizontally polarized probe pulse ( Fig. 1d ) indicates that the mechanical motion from the two phonon modes equals in magnitude and in opposite directions. This interference effect is a signature of two opposite sign perturbations to the plasmonic mode and is critical evidence for our ability to control the detection below the diffraction limit. When the probe polarization is vertical ( Fig. 1f ), the two perturbations are in phase and the interference effect is no longer observed. This measurement indicates a symmetry difference between the lower frequency and higher frequency phonon modes in excellent agreement with the nanomechanical simulations ( Fig. 1b,c ). The numerical calculation for an isolated gold nanostructure indicates antisymmetric and symmetric modes at 8.6 and 12.6 GHz, respectively. The observed splitting of the higher energy resonance is because of substrate effects; in particular, the substrate shifts the resonance frequencies of the modes and breaks the out-of-plane symmetry allowing the excitation of additional out-of-plane modes (see Supplementary Figs 3–6 ). The observed polarization dependence of the phononic response demonstrates that plasmonic nanostructures can selectively detect mechanical displacements. Future applications of this technique can leverage the advances in coherent control of electromagnetic fields to selectively detect phonons on narrow tips [30] and complex nanostructures [31] , revolutionizing the ability to detect phonons in nanoscale regions from the far field. Tailoring the phonon modes via symmetry The polarization manipulation of the probe surface plasmon allows selective detection; manipulating the pump polarization, however, does not allow selective excitation because of energy transport by superdiffusive electrons. The amplitudes of the phonon eigenmodes can be controlled through design of the nanostructures and understanding of the hot electron dynamics. In particular, we use the fact that the phonons are excited because of an isotropic heating to prevent the excitation of antisymmetric modes by designing the structure to be symmetric. As an example, we design a symmetric Swiss-cross and find that only the symmetric mode is excited as seen in Fig. 2a . Similar phonon modes are observed for all pump and probe polarization combinations, illustrating that in a small symmetric structure the phonon modes excited are relatively independent of the pump polarization. The antisymmetric mode is not excited despite the fact that the structure supports symmetric and antisymmetric modes as shown in the numerical model in Fig. 2b . In the numerical analysis, we first assume isotropic heating of the free-standing nanostructure, because of superdiffusive transport effects, and then calculate the resulting expansion of the nanostructure yielding a spatially dependent displacement. We then calculate the relative amplitude of each phonon mode by decomposing the initial displacement profile into the basis of vibrational eigenmodes [32] , [33] . The amplitudes of the two modes when one arm length is fixed and the other varied are shown in Fig. 2b . When the lengths of the arms are equal, we find that the predicted amplitude of the antisymmetric mode is zero, in agreement with experiments. In the limit of high aspect ratio L x >> L y , the antisymmetric mode becomes similar to the extensional mode of a bar, which is efficiently excited. The symmetric mode instead has a low excitation efficiency [32] and approaches a breathing mode. The agreement between the experiments and the model indicates that the lattice heating is relatively uniform for both excitation polarizations. This is consistent with the literature values for the diffusion length of non-equilibrium electrons in gold, the characteristic length over which electrons deposit their kinetic energy, which is ~40 nm (refs 16 , 34 , 35 ). Future experiments on larger structures or structures composed of materials with shorter electron diffusion lengths can be used to study electron transport and their interaction with coherent phonons at the nanoscale. 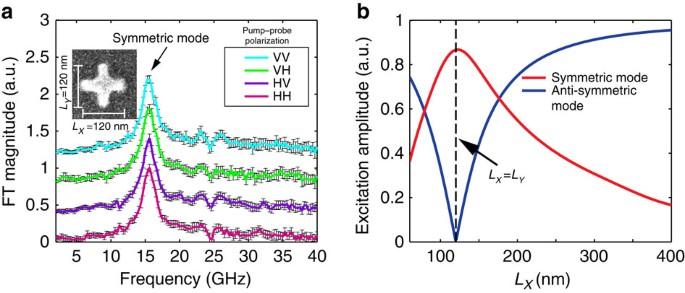Figure 2: Tailoring the phonon modes through nanostructure design. In a symmetric nanostructure only a single phonon mode is observed (a), which is independent of the pump or probe polarization. This is in contrast to the 120 × 90 nm structure (Fig. 1), in which two acoustic eigenmodes, symmetric and antisymmetric, are excited and observed. The error bars are the s.d. of multiple pump–probe experiments. Time traces for parallel and orthogonal pump and probe polarizations are shown inSupplementary Fig. 11. The mechanism behind this effect is a zero overlap between the displacement fields generated by the laser pulse and those of the antisymmetric phonon mode. For a nanostructure small enough to be uniformly heated, this occurs when the nanostructure is symmetric (equal arm lengths). Under the assumption of isotropic heating, the initial amplitudes of the various phonon modes can be controlled through nanostructure design, as calculated for a nanostructure without a substrate inb. Fixing the length of the vertical arm (Ly), the excitation efficiency of the two phonon modes varies as a function of the horizontal arm length (Lx) (b). When the structure is symmetric (Lx=Ly), the antisymmetric mode is not excited, in agreement with experiments. Although not excited, the antisymmetric mode is still an eigenmode of the structure: it is ‘dark’ for this excitation mechanism. In contrast, a highly elongated structure (Lx>>Ly) more efficiently generates the antisymmetric mode. Figure 2: Tailoring the phonon modes through nanostructure design. In a symmetric nanostructure only a single phonon mode is observed ( a ), which is independent of the pump or probe polarization. This is in contrast to the 120 × 90 nm structure ( Fig. 1 ), in which two acoustic eigenmodes, symmetric and antisymmetric, are excited and observed. The error bars are the s.d. of multiple pump–probe experiments. Time traces for parallel and orthogonal pump and probe polarizations are shown in Supplementary Fig. 11 . The mechanism behind this effect is a zero overlap between the displacement fields generated by the laser pulse and those of the antisymmetric phonon mode. For a nanostructure small enough to be uniformly heated, this occurs when the nanostructure is symmetric (equal arm lengths). Under the assumption of isotropic heating, the initial amplitudes of the various phonon modes can be controlled through nanostructure design, as calculated for a nanostructure without a substrate in b . Fixing the length of the vertical arm ( L y ), the excitation efficiency of the two phonon modes varies as a function of the horizontal arm length ( L x ) ( b ). When the structure is symmetric ( L x = L y ), the antisymmetric mode is not excited, in agreement with experiments. Although not excited, the antisymmetric mode is still an eigenmode of the structure: it is ‘dark’ for this excitation mechanism. In contrast, a highly elongated structure ( L x >> L y ) more efficiently generates the antisymmetric mode. Full size image Coherent control of acoustic phonons In order to excite arbitrary acoustic modes, the spatially selective excitation method is less viable because of the fact that our nanostructures are comparable in size to the diffusion length of the electrons; therefore, hot electron superdiffusion will spread energy throughout the structure before the coherent acoustic phonon excitation, regardless of the initial energy distribution. In contrast, temporal coherent control does not require localized heating. Temporal coherent control was originally proposed to manipulate the quantum states of atoms and molecules to yield a desired reaction product [36] . It has since been used to manipulate spin qubits [37] , the near-field of surface plasmons [31] and the vibrational state of single molecules [38] . In phononics, coherent control techniques [39] have been used to selectively excite a specific subset of modes in nanoparticles [40] , [41] and semiconductor superlattices [42] . Complex structures such as the ones studied in this work support a rich spectrum of acoustic eigenmodes and can be potentially used to synthesize arbitrary phonon pulses. In order to control the behaviour of the phonons in the Swiss-cross structures, we generate a pair of excitation pulses (pump and control in Supplementary Fig. 7 ) with a variable temporal separation. We then measure the transient transmission with a probe pulse. Depending on the temporal separation of the two excitation pulses, the phonons can either be enhanced or suppressed. Two excitation pulses spaced in time by an integer number of phonon periods will enhance the mode, while a half integer spacing suppresses the mode by destructive interference. In this way, we can set the initial strain/displacement pattern to be a linear combination of the strain profiles of each eigenmode. The amplitudes of the phonon modes that are excited are shown in Fig. 3a . At zero delay between the pump and control pulses we see all of the modes of the system (trace i, Fig. 3a ). With a properly timed control pulse delay (100 ps), we can make the normally weak antisymmetric mode stronger than the symmetric mode (trace iii, Fig. 3a ). The phononic response for the full set of control pulse delays is shown in Fig. 3c,d . The amplitudes of the modes are shown in Fig. 3d (dots) along with a model in which we assume a phase delayed excitation of the phonon modes (solid line). We take the initial amplitudes from the single pump experiment and predict the amplitudes at different pump-control pulse delays in the coherent control experiment by assuming a coherent addition of the phonons generated by the two pulses. The agreement between the experiment and the model indicates that tailored frequency responses can be predicted and generated using the coherent control of phonons. 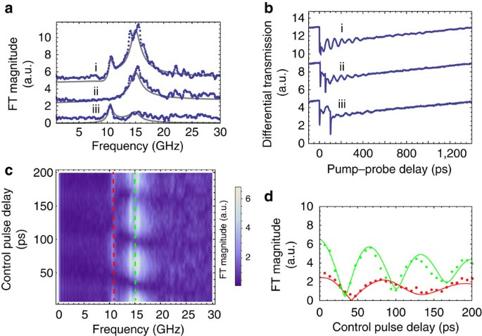Figure 3: Dynamic control of the phonon modes of a Swiss-cross with temporal coherent control. For a designed nanostructure, temporal coherent control can change the phonon modes on demand. (a) In the 120 × 90 nm Swiss-cross structure where both modes are excited (i) pump and control pulses separated by an appropriate time delay can selectively excite the higher frequency symmetric mode (ii) or the lower frequency antisymmetric mode (iii). Without coherent control, both modes are excited (i). The control pulse delay is the delay between the first pump pulse and the second pump pulse. In the transient transmission spectra (b), the two sharp dips are the pump and control pulses that are temporally separated by the control pulse delay. The phonon spectra i, ii and iii are produced with pump-control pulse delays of 5, 46 and 100 ps. The amplitude as a function of frequency and pump-control pulse delay is shown inc, with specific traces corresponding to the symmetric (green dots) and antisymmetric modes (red dots) are shown ind. The parameters for the calculation (solid line) are derived from the fit of the 5-ps control pulse delay pump experiment (grey curve i ina) with the fit function inSupplementary Note 1. Figure 3: Dynamic control of the phonon modes of a Swiss-cross with temporal coherent control. For a designed nanostructure, temporal coherent control can change the phonon modes on demand. ( a ) In the 120 × 90 nm Swiss-cross structure where both modes are excited (i) pump and control pulses separated by an appropriate time delay can selectively excite the higher frequency symmetric mode (ii) or the lower frequency antisymmetric mode (iii). Without coherent control, both modes are excited (i). The control pulse delay is the delay between the first pump pulse and the second pump pulse. In the transient transmission spectra ( b ), the two sharp dips are the pump and control pulses that are temporally separated by the control pulse delay. The phonon spectra i, ii and iii are produced with pump-control pulse delays of 5, 46 and 100 ps. The amplitude as a function of frequency and pump-control pulse delay is shown in c , with specific traces corresponding to the symmetric (green dots) and antisymmetric modes (red dots) are shown in d . The parameters for the calculation (solid line) are derived from the fit of the 5-ps control pulse delay pump experiment (grey curve i in a ) with the fit function in Supplementary Note 1 . Full size image In conclusion, we have demonstrated optical manipulation and detection of the gigahertz mechanical motion of complex nanostructures using multimodal phonon interference effects. We observe optically the polarization-dependent interference of the symmetric and antisymmetric phonon modes. In addition, through coherent control and structure design we can tailor which modes are excited by the plasmonically generated superdiffusive electrons. Plasmonic nanostructures may expand the toolbox of phononics techniques [43] , [44] at the nanoscale. The presented results open new routes for the development of coherent phonon sources and are a step towards the realization of nanophononic devices capable of probing electronic, thermal and phononic states. Optical measurements The pump is generated by a titanium–sapphire femtosecond laser (Mai Tai HP, 820 nm, ~100 fs) with a power of 4 mW and the probe is from an optical parametric oscillator (Inspire, 700 nm, ~100 fs, <1 mW) pumped with the same laser. The repetition rate of both systems is 80 MHz. The pump and probe beams are collinear and are focused with a 0.25 NA objective and collected with a 0.65 NA objective. The pump and probe beam waists are 5 μm. Spectral filters are used to separate the pump and probe before detection. The analysis procedure for the transient transmission measurements is illustrated in Supplementary Fig. 8 . Numerical simulations The phonon dynamics are simulated using the finite element solver COMSOL Multiphysics. We calculate, in the frequency domain, the response of a nanoparticle to an impulse strain in the metal because of the pulsed laser excitation. The thermal strain generates a force that sets the particle in motion. Given the mechanical motion, we take a simple model for the detection by the plasmon and assume that the transient transmission change will be proportional to the change in length. As an example, we calculate the response, in the frequency domain, of a 40-nm-radius gold nanoparticle to an impulse strain in the metal because of the pulsed laser excitation. The thermal strain generates a force that sets the particle in motion. The phonon dynamics can be calculated by solving Navier’s equation, which governs linear elastodynamics in an isotropic medium: where λ and μ are Lamé’s first and second parameters, ρ is the density, u is the displacement vector, F is the force generated by the thermal strain in the metal, ε thermal = α Δ T , and α is the coefficient of thermal expansion. We solve this equation in the frequency domain with continuity of displacement and stress at the interface between materials. We now sketch out the solution for a model system: a spherical gold nanoparticle in an infinite glass matrix as shown in Supplementary Fig. 9b . With spherical symmetry, Navier’s equation simplifies to [45] : where ν p is the longitudinal (p-wave) speed of sound and F r ( ω ) is the radial force in the frequency domain for a thermal strain [46] : F r ( ω )=(3 λ +2 μ ) α Δ T . We solve for the displacement as a function of frequency and position analytically and with the finite element method using COMSOL Multiphysics. We see excellent agreement between the two methods for the radial displacement magnitude ( Supplementary Fig. 9b ) as a function of frequency at the surface of the sphere. In addition, we see excellent agreement in the displacement as a function of the distance from the centre of the sphere at the resonance frequency ( Supplementary Fig. 9c ). The region inside of the nanoparticle is highlighted in gold and the glass is coloured blue. The oscillations in the glass indicate acoustic energy flow away from the particle. We note that the materials were considered to be lossless and both methods show a broad resonance ( Q ~10) because of radiation damping. For the finite element method simulations, we use a perfectly matched layer to simulate an infinite medium. The material parameters used in the calculations are listed in Supplementary Table 1 . For the Swiss-Cross nanostructures, an analytic solution is not available; therefore, we use the finite element method to simulate the dynamics. How to cite this article: O’Brien, K. et al . Ultrafast acousto-plasmonic control and sensing in complex nanostructures. Nat. Commun. 5:4042 doi: 10.1038/ncomms5042 (2014).